Fine-tuned local coordination environment of Pt single atoms on ceria controls catalytic reactivity Constructing single atom catalysts with fine-tuned coordination environments can be a promising strategy to achieve satisfactory catalytic performance. Herein, via a simple calcination temperature-control strategy, CeO 2 supported Pt single atom catalysts with precisely controlled coordination environments are successfully fabricated. The joint experimental and theoretical analysis reveals that the Pt single atoms on Pt 1 /CeO 2 prepared at 550 °C (Pt/CeO 2 -550) are mainly located at the edge sites of CeO 2 with a Pt–O coordination number of ca . 5, while those prepared at 800 °C (Pt/CeO 2 -800) are predominantly located at distorted Ce substitution sites on CeO 2 terrace with a Pt–O coordination number of ca . 4. Pt/CeO 2 -550 and Pt/CeO 2 -800 with different Pt 1 -CeO 2 coordination environments exhibit a reversal of activity trend in CO oxidation and NH 3 oxidation due to their different privileges in reactants activation and H 2 O desorption, suggesting that the catalytic performance of Pt single atom catalysts in different target reactions can be maximized by optimizing their local coordination structures. In recent years, different types of single atom catalysts have been applied in many energy and environment-related reactions because of their maximum atomic utilization efficiency, unique electronic states, or higher stability comparing to the nano-cluster/particle catalysts [1] , [2] , [3] , [4] , [5] , [6] , [7] . With the deepening of research in this area, it has been revealed that the performance of single atom catalysts on specified supports for certain reactions such as thermal catalysis and electrocatalysis could be significantly promoted by tuning their oxidation states or coordination environments [8] , [9] , [10] , [11] , [12] , [13] , [14] . Among these single atom catalytic materials, the Pt single atom (Pt 1 ) catalyst supported on rare earth metal oxide CeO 2 is one of the most popular catalyst systems, which has been studied extensively for the elimination of environmental pollutants and energy conversion [15] , [16] , [17] , [18] , [19] . Most recently, various synthesis methods have been employed to fabricate Pt single atoms with improved catalytic performance [18] , [19] , [20] . For instance, by creating stable hydroxyl groups on Pt 1 /CeO 2 catalyst using hydrothermal treatment at 750 °C, the CO oxidation activity on Pt 1 /CeO 2 could be enhanced dramatically [20] . Ma et al. reported that modulating Pt 1 /CeO 2 with phosphate (PO 4 3− ) could increase the valence state of Pt and facilitate the reactant adsorption and hydrogen spillover, which accordingly boosted the catalytic activity for styrene hydrogenation [21] . Jeong et al. tuned the oxidation state of Pt single atoms on CeO 2 using hydrogen reduction method for maximizing the catalytic activity in CO, CH 4 , and NO oxidation [22] . Meanwhile, many experimental and theoretical efforts have been devoted to synthesizing Pt 1 catalysts on CeO 2 support with optimal coordination environment or constructing reasonable Pt 1 –CeO 2 structural models, which could help better understand the reaction mechanisms and reveal the origin of different catalytic performances on Pt single atom catalysts [23] , [24] , [25] , [26] , [27] , [28] . For example, Jiang et al. successfully synthesized a Pt 1 /CeO 2 catalyst with asymmetric Pt 1 –O 4 configuration, which exhibited much higher CO oxidation activity than the reference catalyst with symmetric Pt 1 –O 4 configuration [27] . Wang et al. reported that CO–Pt 1 –O 3 was the dominant configuration for CO adsorption on Pt 1 catalyst supported on oxygen plasma-pretreated CeO 2 , and such Pt 1 species exhibited higher CO oxidation activity and better resistance towards sintering comparing to that in conventional Pt 1 /CeO 2 catalyst [28] . So far, no comprehensive work has been reported focusing on the precise tuning of local coordination environment for Pt single atoms on CeO 2 support to modulate their activity in different catalytic reactions and at the same time revealing the intrinsic structure-activity relationships. Herein, we proposed a simple strategy for fine-tuning the exact location of Pt single atoms by controlling the calcination temperature of Pt/CeO 2 catalysts prepared by the facile incipient wetness impregnation (IWI) method. The Pt single atoms on Pt 1 /CeO 2 catalysts calcined at different temperatures could have different coordination environments. Through systematic experimental characterizations, catalytic performance testing, and density functional theory (DFT) based simulations of Pt 1 /CeO 2 catalysts, it was clearly revealed that the CeO 2 -supported Pt single atoms with fine-tuned local coordination structures could exhibit strikingly distinct catalytic behaviors in different oxidation reactions such as CO oxidation versus NH 3 oxidation, which needs to be taken into consideration for practical applications of single atom catalysis in the future. Constructing Pt 1 with different coordination environments To minimize the potential structural change of pure CeO 2 support after the deposition of Pt followed by calcination, the CeO 2 used in this work was pre-calcined in air at 800 °C for 12 h to obtain pre-stabilized structure. Moreover, the deposition of Pt was reported to have a positive effect on stabilizing the CeO 2 support [29] . As shown in Supplementary Fig. 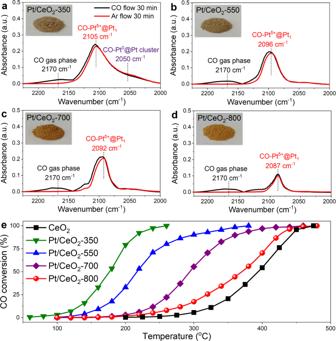Fig. 1: Pt status determined by CO adsorption and corresponding CO oxidation activity. In situ DRIFTS of CO adsorption at 25 °C onaPt/CeO2-350,bPt/CeO2-550,cPt/CeO2-700 anddPt/CeO2-800 (inserted are the photos of different catalysts);eCO oxidation performance on Pt/CeO2-350, Pt/CeO2-550, Pt/CeO2-700 and Pt/CeO2-800 (Reaction condition: [CO] = [O2] = 1%, balanced with Ar, WHSV = 400,000 mL∙gcat−1∙h−1). 1 and Table 1 , the pure CeO 2 support and CeO 2 supported Pt catalysts showed almost the same specific surface area and pore structure, suggesting no obvious change in the textural structure of CeO 2 support during the catalyst fabrication process. Table 1 Textural properties determined by N 2 physisorption results, band gap determined by UV–Vis spectra, and the average valence states of Pt species determined by XANES linear combination fitting Full size table To determine the states of Pt species on Pt/CeO 2 catalysts, in situ DRIFTS of CO adsorption at 25 °C was first performed (Fig. 1 ). The IR bands assigned to CO adsorbed on ionic Pt single sites (CO-Pt δ+ @Pt 1 ) were observed on all four catalysts at 2087–2105 cm −1 . For Pt/CeO 2 -350, a broad band at ca . 2050 cm −1 ascribed to CO adsorbed on metallic Pt sites from Pt clusters (CO-Pt 0 @Pt clusters) was also detected. Although the Pt species on Pt/CeO 2 -550, Pt/CeO 2 -700, and Pt/CeO 2 -800 were mainly in the form of single atoms, the monotonical redshift of CO-Pt δ+ @Pt 1 band as the calcination temperature increased indicated the different local coordination environments or oxidation states of Pt single atoms. As concluded from previous works, the center of the IR band assigned to CO linearly adsorbed on Pt 1 supported by CeO 2 usually ranged between 2085 and 2105 cm −1 [24] , [27] , [30] , [31] . The 9 cm −1 redshift of IR band (from 2096 to 2087 cm −1 ) for CO adsorption as the calcination temperature increased from 550 to 800 °C could be considered as a significant change, indicating the remarkably distinct Pt 1 local structures on Pt/CeO 2 -550 and Pt/CeO 2 -800. Moreover, the Pt/CeO 2 catalysts calcined at different temperatures showed varied colors (from dark brown to golden brown), suggesting the different states of Pt 1 species as well (inserted photos in Fig. 1a–d ). Fig. 1: Pt status determined by CO adsorption and corresponding CO oxidation activity. In situ DRIFTS of CO adsorption at 25 °C on a Pt/CeO 2 -350, b Pt/CeO 2 -550, c Pt/CeO 2 -700 and d Pt/CeO 2 -800 (inserted are the photos of different catalysts); e CO oxidation performance on Pt/CeO 2 -350, Pt/CeO 2 -550, Pt/CeO 2 -700 and Pt/CeO 2 -800 (Reaction condition: [CO] = [O 2 ] = 1%, balanced with Ar, WHSV = 400,000 mL∙g cat −1 ∙h −1 ). Full size image CO oxidation is a commonly used probe reaction to evaluate the catalytic oxidation performance of Pt–CeO 2 -based catalysts and many other catalyst systems [32] , [33] , [34] . In turn, the difference in the local structure of Pt–CeO 2 catalysts can be reflected by their corresponding CO oxidation activity [27] , [35] . As demonstrated in Fig. 1e , with the increase of calcination temperature, the CO oxidation activity on Pt/CeO 2 catalysts decreased monotonically. The presence of Pt clusters on Pt/CeO 2 -350 (Fig. 1a ) well explained its best CO oxidation activity, as the Pt cluster-CeO 2 interfacial sites were considered as the most active species for CO oxidation [30] , [36] , [37] , [38] . Although the Pt species on Pt/CeO 2 -550, Pt/CeO 2 -700, and Pt/CeO 2 -800 were all in Pt single atom form, the significant difference in the CO oxidation activity on Pt/CeO 2 -550, Pt/CeO 2 -700, and Pt/CeO 2 -800 revealed that the Pt single atoms with varied states were successfully created on these three catalysts. H 2 -TPR technique is a powerful tool to evaluate the dispersion of Pt species as well as the strength of Pt-O-Ce interaction on Pt/CeO 2 based catalysts [39] , [40] . Herein, the H 2 -TPR profiles of Pt/CeO 2 -550, Pt/CeO 2 -700, Pt/CeO 2 -800 were collected to investigate the interaction between Pt single atoms and CeO 2 support (Fig. 2a, b ). The H 2 -consumption peaks centered around 150 °C could be attributed to the reduction of Pt–O–Ce structure, while the H 2 -consumption peaks at ca . 420 and 785 °C could be ascribed to the reduction of surface Ce 4+ species and bulk CeO 2 , respectively [41] . Interestingly, as the calcination temperature increased from 550 to 800 °C, the H 2 -consumption peak assigned to the reduction of Pt–O–Ce structure shifted to higher temperatures (126 °C → 173 °C) with enhanced intensity, indicating the different strength of Pt–O–Ce interaction as well as the different locations of Pt single atoms on Pt/CeO 2 -X catalysts. For Pt/CeO 2 -700, the Pt singe atoms should be in a mixed state of the Pt species in Pt/CeO 2 -550 and Pt/CeO 2 -800. Based on the CO oxidation evaluation results, Pt/CeO 2 -800 catalyst showed very similar CO oxidation activity to the pure CeO 2 support. Therefore, the much more intensive H 2 -consumption peak of Pt–O–Ce species at higher reduction temperature on Pt/CeO 2 -800 suggested that the Pt single atoms on this catalyst might have migrated into the surface lattice of CeO 2 support and the isolated Pt atoms were strongly bonded to CeO 2 through more Pt–O–Ce linkages. Fig. 2: Pt-CeO 2 interaction determined by H 2 -TPR and UV–Vis spectra. a , b H 2 -TPR profiles for Pt/CeO 2 -X catalysts; c UV–Vis spectra of CeO 2 support and Pt/CeO 2 -X catalysts; d the plots of ( αhv ) 2 vs. photon energy ( hv ) for CeO 2 support and Pt/CeO 2 -X catalysts (X = 550, 700 and 800). Full size image UV–Vis spectroscopy analysis was also conducted to study the interaction between Pt single atoms and CeO 2 support. As shown in Fig. 2c , the band below 400 nm on CeO 2 and Pt/CeO 2 -X catalysts (X = 550, 700, and 800) could be attributed to the charge transfer for O 2p → Ce 4f transition [42] . Interestingly, after the deposition of Pt, an additional strong absorption assigned to the absorption tail or Urbach tail was observed at 400–600 nm, which was related to the band gap smearing induced by defect accumulation [43] . For Pt/CeO 2 -X catalysts, such absorption tail could be due to the structural disorders induced by the highly dispersed Pt species. Moreover, with the increase of the calcination temperature, the absorption intensity at 400–600 nm enhanced accordingly, suggesting that the Pt/CeO 2 catalyst calcined at higher temperature possessed higher surface structural disorder and more surface defects, possibly resulted from the migration of Pt single atoms into CeO 2 lattice and the stronger interaction between Pt and CeO 2 support [44] , [45] . The formation of more surface defects on Pt/CeO 2 -800 was further confirmed by the in situ DRIFTS of methanol adsorption experiments (Supplementary Fig. 2 ), in which the band at 1034 cm −1 assigned to bridging methoxy species on two Ce 4+ cations with an oxygen vacancy on Pt/CeO 2 -800 showed much higher intensity than that on pristine CeO 2 and Pt/CeO 2 -550 [46] . The indirect band gap was also calculated by Davis and Mott equation for further understanding the interaction between Pt species and CeO 2 support within Pt/CeO 2 -X catalysts (Fig. 2d and Table 1 ) [43] , [47] . The band gap for Pt/CeO 2 -X catalysts was much lower than that for CeO 2 support (3.23 eV), indicating the insertion of metal levels between the valence and conduction bands of CeO 2 as well as the strong interaction through Pt–O–Ce linkage [48] . The lower band gap for Pt/CeO 2 -800 (2.61 eV) than those for Pt/CeO 2 -550 (2.96 eV) and Pt/CeO 2 -700 (2.80 eV) well supported the viewpoint that stronger Pt–O–Ce interaction was formed on Pt/CeO 2 -800 catalyst. Location and coordination environment of Pt single atoms AC-HAADF-STEM images of Pt/CeO 2 -550 and Pt/CeO 2 -800 were collected to determine the location of Pt species (Fig. 3 ). CeO 2 support was found to selectively expose (110) crystal plane. As expected, no identifiable Pt clusters were found on Pt/CeO 2 -550 and Pt/CeO 2 -800, and only bright dots assigned to isolated Pt atoms were observed. It was also shown by the high-resolution EDS mapping results that the Pt species were in highly dispersed state on both Pt/CeO 2 -550 and Pt/CeO 2 -800 (Supplementary Fig. 3 ). Moreover, the isolated Pt single atoms on both catalysts were found to fit well into the Ce columns on CeO 2 (110) plane. Based on the results of in situ DRIFTS of CO adsorption, CO oxidation activity evaluation, H 2 -TPR and UV–Vis spectra, it could be deduced that the Pt single atoms on Pt/CeO 2 -550 and Pt/CeO 2 -800 should be in different status including the locations and coordination environments. Considering that the AC-HAADF-STEM images were just projection drawings, the Pt single atoms on Pt/CeO 2 -550 and Pt/CeO 2 -800 could be located at different substitution sites or epitaxial growth sites of Ce on CeO 2 support, which enabled the Pt single atoms to be in different status but all observed in the Ce columns on CeO 2 (110) plane. With the aid of line profiles of AC-HAADF-STEM images (Fig. 3a, b and Supplementary Fig. 4 ), the different locations of Pt single atoms on Pt/CeO 2 -550 and Pt/CeO 2 -800 could be well discerned. For Pt/CeO 2 -550, the Pt atoms were mainly located at the edge or step sites on the surface of CeO 2 , while the Pt atoms on Pt/CeO 2 -800 were possibly located at the Ce substitution sites on the CeO 2 terrace (e.g., embedded into the surface lattice of CeO 2 ). Fig. 3: Location of Pt single atoms on CeO 2 . AC-HAADF-STEM images and the line profiles of a Pt/CeO 2 -550 and b Pt/CeO 2 -800 (additional line profiles of Pt/CeO 2 -800 can be found in Supplementary Fig. 4 ). In situ XRD patterns for c Pt/CeO 2 -550 and d Pt/CeO 2 -800; e the refined lattice parameters of Pt/CeO 2 (without calcination), standard CeO 2 , Pt/CeO 2 -550 and Pt/CeO 2 -800 obtained by Rietveld refinements. Full size image To further reveal the location of Pt atoms on CeO 2 support, two sets of in situ XRD experiments were designed, in which the XRD patterns were collected continuously throughout the sample heating (to 550 or 800 °C) and cooling process (Supplementary Fig. 5 and Fig. 3c, d ). Before the measurements, the CeO 2 powder newly impregnated with Pt nitrate solution was dried in air at 120 °C for 30 min to remove excess H 2 O (denoted as Pt/CeO 2 ). During the calcination process to obtain Pt/CeO 2 -550, the XRD peaks shifted to lower angles in the heating stage from RT to 550 °C, and shifted back to higher angles in the cooling stage, which should be related to the lattice expansion and lattice contraction, respectively [49] . During the calcination process to obtain Pt/CeO 2 -800, the XRD peaks also shifted to lower angles in the heating stage (< 620 °C) due to the lattice expansion of CeO 2 as well. However, an abrupt shift of XRD peaks back to high angles was observed for Pt/CeO 2 -800 at higher temperature of ca . 620 °C, which should be resulted from the desorption of O 2 to form surface Ce 2 O 3 species at elevated temperatures [50] . The XRD peaks for bare CeO 2 support showed a similar shift trend during the heating and cooling stages as those for Pt/CeO 2 -550 and Pt/CeO 2 -800 catalysts (Supplementary Fig. 6 ). After calcination at 550 and 800 °C, the XRD diffraction peaks of Pt/CeO 2 catalysts shifted to higher angles in varying degrees. Considering that the CeO 2 support has already been pre-stabilized by calcination at 800 °C for 12 h, the shift in the diffraction peaks of Pt/CeO 2 should be due to the lattice expansion or contraction of CeO 2 induced by Pt species [51] . By conducting the Rietveld refinements of XRD patterns for Pt/CeO 2 , Pt/CeO 2 -550, and Pt/CeO 2 -800, the refined lattice parameters of CeO 2 on these samples were calculated (Fig. 3e ). It was noticeable that the lattice parameter of uncalcined Pt/CeO 2 and Pt/CeO 2 -550 was slightly higher than that of standard CeO 2 reference, which should result from the perturbation effect of Pt deposition on CeO 2 surface. Interestingly, when the calcination temperature increased to 800 °C, a dramatic decrease in the lattice parameter was observed, which might be related to the substitution of Ce ions by Pt ions with smaller ionic radius (Ce 4+ = 0.970 Å, Ce 3+ = 1.280 Å, Pt 4+ = 0.625 Å, Pt 2+ = 0.800 Å) and further distortion [43] , [52] , in line with the previous report that the Pt 2+ might diffuse into CeO 2 lattice during the high temperature calcination process [43] . The in situ XRD results further suggested that the Pt atoms might have been incorporated into the surface lattice on CeO 2 terrace within Pt/CeO 2 -800 catalyst. X-ray absorption spectroscopy (XAS) analysis was conducted to further elucidate the valence states and the coordination environments of Pt single atoms on Pt/CeO 2 -X catalysts. As shown in Fig. 4a and Supplementary Fig. 7a , the white line (the intense absorption in the near-edge region) intensities of Pt-L 3 XANES for the Pt/CeO 2 catalysts were always much higher than that for Pt foil but lower than that for PtO 2 , indicating the intermediate valence state of Pt species between 0 and +4 on Pt/CeO 2 -X catalysts. Interestingly, the white line intensity of Pt-L 3 XANES on Pt/CeO 2 catalysts decreased monotonically as the calcination temperature increased, indicating the decreased Pt valence state accordingly. The XANES linear combination fitting was performed to further determine the average valence state of Pt species (Supplementary Fig. 8 , Table 1 and Supplementary Table 1 ). 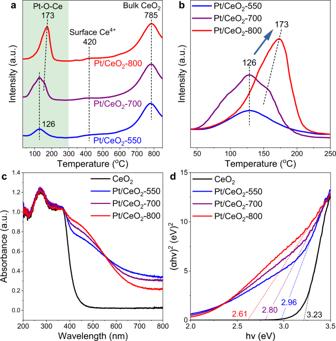Fig. 2: Pt-CeO2interaction determined by H2-TPR and UV–Vis spectra. a,bH2-TPR profiles for Pt/CeO2-X catalysts;cUV–Vis spectra of CeO2support and Pt/CeO2-X catalysts;dthe plots of (αhv)2vs. photon energy (hv) for CeO2support and Pt/CeO2-X catalysts (X = 550, 700 and 800). As expected, the Pt species on Pt/CeO 2 -800 indeed showed much lower valence state (2.7 ± 0.1) than those on Pt/CeO 2 -550 (3.4 ± 0.1), which was further supported by the Pt 4f XPS results that more Pt 2+ species were created on Pt/CeO 2 -800 comparing to those on Pt/CeO 2 -550 (Supplementary Table 2 and Supplementary Fig. 9 ). Fig. 4: Coordination environment of Pt single atoms determined by XAS analysis. a Normalized XANES and b EXAFS magnitude of the Fourier transformed k 2 -weighted χ( k ) data for Pt/CeO 2 -550 (blue) and Pt/CeO 2 -800 (red) at the Pt-L 3 edge. Pt foil (orange) and PtO 2 (black) references were used for XANES linear combination fitting and EXAFS comparison. c Three possible geometries of Pt single atoms at the edge or step sites on CeO 2 (110) within Pt/CeO 2 -550. d The reconstruction of Pt single atoms on CeO 2 (110) terrace from six-coordination sites to square-planar like coordination sites within Pt/CeO 2 -800. Full size image Herein, to further reveal the local coordination structure of Pt single atoms on Pt/CeO 2 -550 and Pt/CeO 2 -800 catalysts, the EXAFS curve fitting was conducted and the results are plotted in both R space and k space (Fig. 4b , Supplementary Fig. 7b , Supplementary Fig. 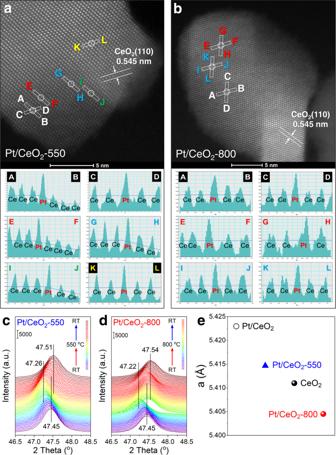Fig. 3: Location of Pt single atoms on CeO2. AC-HAADF-STEM images and the line profiles ofaPt/CeO2-550 andbPt/CeO2-800 (additional line profiles of Pt/CeO2-800 can be found in Supplementary Fig.4). In situ XRD patterns forcPt/CeO2-550 anddPt/CeO2-800;ethe refined lattice parameters of Pt/CeO2(without calcination), standard CeO2, Pt/CeO2-550 and Pt/CeO2-800 obtained by Rietveld refinements. 10 and Supplementary Table 3 ). The absence of Pt–O–Pt and Pt–Pt coordination shells and the exclusive observation of Pt–O and Pt–O–Ce coordination shells further evidenced the formation of Pt single atoms on Pt/CeO 2 -550 and Pt/CeO 2 -800. Although Pt/CeO 2 -800 indeed showed a lower coordination number (CN) of Pt–O (CN Pt– O = 4.4 ± 0.3) than Pt/CeO 2 -550 (CN Pt– O = 5.1 ± 0.4), a higher CN of Pt–O–Ce was observed on Pt/CeO 2 -800 (CN Pt– O– Ce = 4.2 ± 0.3) comparing to that on Pt/CeO 2 -550 (CN Pt– O– Ce = 3.7 ± 0.3), further validating the formation of more Pt–O–Ce linkages within Pt/CeO 2 -800, which could be further proved by Raman spectra (Supplementary Fig. 11 ). As discussed above, for Pt/CeO 2 -550, the Pt single atoms should be mainly located at the edge or step sites of CeO 2 (110), which did not induce any lattice shrinkage of CeO 2 (Fig. 4c ). In contrast, for Pt/CeO 2 -800, the significant lattice shrinkage of CeO 2 support could be related to the incorporation of Pt atoms into the surface lattice of CeO 2 (110). For Pt atoms substituting the surface Ce sites on CeO 2 (110) in an ideal model, the CN Pt– O should be 6, which was higher than the CN Pt– O on Pt/CeO 2 -800 (CN Pt– O = 4.4 ± 0.3). However, since Pt 2+ species possessed smaller ionic radius ( ca . 0.800 Å) than Ce 4+ ( ca . 0.970 Å), a significant reconstruction of Pt single atoms from six-coordination sites to square-planar like coordination sites could occur on Pt/CeO 2 -800 to balance the space and charge, thus leading to the decrease in the CN Pt– O from 6 to 4 (Fig. 4d and Supplementary Fig. 12 ). Similar reconstruction of Pt single atoms was also reported to occur on CeO 2 (111) [26] . DFT calculations on the coordination environment of Pt 1 To confirm the conjecture about the location, as well as the coordination environment of Pt single atoms on Pt/CeO 2 -550 and Pt/CeO 2 -800, DFT calculations were performed. For Pt/CeO 2 -550, based on the experimental evidence showing that Pt single atoms were mainly located at or near the edge/step sites on CeO 2 (110) surface, ten configurations were proposed (Fig. 5a1–a10 and Supplementary Fig. 13 ). Among them, five configurations in which one Ce atom at the edge sites was replaced by one Pt atom were constructed (Fig. 5a1–a5 ). In Pt@CeEdge configuration, Pt replaced Ce atom at the edge sites and coordinated with 6 oxygen atoms to form octahedral Pt–O 6 (Fig. 5a1 and Supplementary Fig. 13a ). Once one or two O atoms on Pt@CeEdge were removed, the Pt@CeEdge configuration evolved into Pt@CeEdge-O or Pt@CeEdge-2O (Fig. 5a2–a3 and Supplementary Fig. 13b, c ), in which Pt coordinated with 5 or 4 oxygen atoms to form Pt–O 5 or square planar Pt–O 4 , respectively. Further removal of another oxygen atom led to the formation of Pt@CeEdgeO v (1) (Fig. 5a4 and Supplementary Fig. 13d ) or Pt@CeEdgeO v (2) (Fig. 5a5 and Supplementary Fig. 13e ) with a Pt–O 3 coordination. Furthermore, another five configurations where Pt atoms located at or near the step sites were constructed. In the configuration of Pt@Step, Pt atom was adsorbed at the step on CeO 2 (110) surface with a Pt–O 4 coordination (Fig. 5a6 and Supplementary Fig. 13f ). Similar to Pt@CeEdge configuration, as shown in Fig. 5a7–a9 and Supplementary Fig. 13g–i , after adding or removing O atoms, three new configurations were obtained (Pt@Step+O, Pt@StepO v (1) and Pt@StepO v (2) ). One configuration in which Pt replaced Ce step atom (Pt–O 4 coordination) was also proposed (Fig. 5a10 and Supplementary Fig. 13j ). Fig. 5: Determination of Pt 1 configurations on CeO 2 through DFT calculations. The formation energy ( E form ) of the considered Pt 1 configurations on CeO 2 (110) under different conditions, i.e., low-temperature (Low T) calcination condition (550 °C, 0.21 atm O 2 pressure), high-temperature (High T) calcination condition (800 °C, 0.21 atm O 2 pressure), and CO adsorption condition (25 °C, 10 −20 atm O 2 pressure) within a Pt/CeO 2 -550 and b Pt/CeO 2 -800. The insert figures are the top view of considered configurations of isolated Pt atoms at or near the edge/step sites on CeO 2 (110) surface within Pt/CeO 2 -550 ( a1 − 10 ), and at the Ce substitution sites of CeO 2 (110) surface within Pt/CeO 2 -800 ( b1 − 10 ). Large yellow, medium blue, and small red balls represented Ce, Pt, and O atoms. Full size image To compare the relative stability of the Pt structures, the formation energy of the above-mentioned configurations was calculated under two different conditions, i.e., calcination condition (550 °C, 0.21 atm O 2 pressure) and condition at which the CO adsorption experiments were performed (25 °C, 10 −20 atm O 2 pressure). As illustrated in Fig. 5a , the formation energies of each configuration under the two conditions were similar, suggesting that the Pt 1 /CeO 2 structures were almost the same after calcination and during CO adsorption process. Furthermore, other than Pt@CeEdge and Pt@CeStep, the rest eight configurations showed low formation energy, suggesting that the isolated Pt atoms could be stably anchored at edge or step sites on CeO 2 (110) with different possible O-coordination environments. For Pt/CeO 2 -800, based on the characterization results indicating that Pt atoms substituted the surface Ce sites on CeO 2 (110), ten configurations of Pt 1 on CeO 2 (110) terrace were proposed (Fig. 5b and Supplementary Fig. 14 ). The most trivial configuration was the one in which Pt substituted Ce on the CeO 2 (110) surface without any change in the arrangement of O atoms (Fig. 5b1 and Supplementary Fig. 14a ), forming an asymmetrical Pt–O 5 -like coordination (Pt@Ce). However, the Pt–O 5 structure could transform to a distorted configuration of Pt@CeDis (1) without enforcing symmetry during the ionic relaxation process (Fig. 5b2 and Supplementary Fig. 14b ), thus forming a Pt–O 4 planar type of coordination. Two other distorted configurations (Pt@CeDis (2) and Pt@CeDis (3) ) were also considered. Pt@CeDis (2) was similar to Pt@CeDis (1) with an O atom displaced towards the top of Pt to form Pt–O 5 configuration (Fig. 5b3 and Supplementary Fig. 14c ). In Pt@CeDis (3) configuration, an O atom was displaced towards a nearby O atom to form O 2 species (Fig. 5b4 and Supplementary Fig. 14d ), yielding a configuration similar to the one suggested by Tang et al. [25] . By adding an additional O atom on top of Pt in Pt@Ce and Pt@CeDis, two configurations of Pt@Ce+O (Fig. 5b5 and Supplementary Fig. 14e ) and Pt@CeDis+O (Fig. 5b6 and Supplementary Fig. 14f ) were achieved, with the formation of Pt–O 6 coordination and Pt–O 5 coordination, respectively. When one O atom was removed from Pt@CeDis, two configurations with O vacancies nearby Pt atoms were constructed, referred as Pt@CeO v (1) (Fig. 5b7 and Supplementary Fig. 14g ) and Pt@CeO v (2) (Fig. 5b8 and Supplementary Fig. 14h ), thus forming Pt–O 4 coordination and Pt–O 3 coordination, respectively. The further removal of one O atom from Pt@CeO v (1) and Pt@CeO v (2) would result in the formation of configurations with two O vacancies, which were denoted as Pt@Ce2O v (1) (Fig. 5b9 and Supplementary Fig. 14i ) and Pt@Ce2O v (2) (Fig. 5b10 and Supplementary Fig. 14j ), respectively. The formation energy of the above-mentioned configurations was also calculated under both calcination condition and CO adsorption condition (Fig. 5b ). Pt@CeDis (1) , Pt@CeDis (3) , Pt@CeO v (1) and Pt@Ce2O v (1) showed the lowest formation energy among the ten configurations. Furthermore, the Pt atoms in these four configurations were in Pt–O 4 coordination. According to the results of H 2 -TPR, Raman spectra, and XAS analysis, the CN Pt– O on Pt/CeO 2 -550 was higher than that on Pt/CeO 2 -800 (5.1 vs. 4.4). Thus, the Pt 1 species on Pt/CeO 2 -550 should be in Pt–O 4+ x ( x > 0) coordination, and the dominant Pt 1 /CeO 2 configuration within Pt/CeO 2 -550 could be Pt@CeEdge-O or Pt@Step+O with CN Pt– O of 5. It is noteworthy that, because of the large difference in chemical potential of oxygen (−0.41 eV) between High T calcination condition and CO oxidation condition, there was noticeable difference in the formation energy of Pt 1 under the two conditions, except for the cases with two oxygen vacancies (Fig. 5b9–b10 ) in which the Pt 1 formation energy was independent of oxygen chemical potential. In contrast, there was virtually no difference in the chemical potential of oxygen (−0.08 eV) between Low T calcination condition and CO oxidation condition, resulting in the virtually identical Pt 1 formation energy under the two conditions (Fig. 5a ). To confirm the Pt 1 /CeO 2 configurations within Pt/CeO 2 -550 and Pt/CeO 2 -800, CO adsorption calculations were conducted. As shown in Supplementary Fig. 15a , for Pt@CeEdge-O within Pt/CeO 2 -550, CO picked up an O atom to form CO 2 during structural (ionic) relaxation, thus forming the configuration of Pt@CeEdge-2O. CO adsorbed on Pt@CeEdge-2O showed a stretching frequency of 2047 cm −1 , with a binding energy ( E B ) of −0.36 eV. When CO picked up another O atom, CO-Pt@CeEdgeO v (1) ( E B = −1.99 eV) or CO-Pt@CeEdgeO v (2) ( E B = −2.17 eV) was formed, which showed stretching frequencies of 2006 and 1949 cm −1 , respectively (Supplementary Fig. 15b, c ). Similar to the case of Pt@CeEdge-O, CO adsorption would pick up an O atom on Pt@Step+O to form Pt@Step (Supplementary Fig. 15d ). CO-Pt@Step showed a stretching frequency of 2012 cm −1 ( E B = −0.38 eV). Further removal of another O atom on CO-Pt@Step resulted in the formation of CO-Pt@StepO v (1) ( E B = −1.99 eV) and CO-Pt@StepO v (2) ( E B = −2.34 eV), showing stretching frequencies of 2012 and 1921 cm −1 , respectively (Supplementary Fig. 15e, f ). For Pt/CeO 2 -800, it was found that CO could not bind on the Pt atom in Pt@CeDis (1) , but could bind on the Ce atom adjacent to Pt atom ( E B = −0.39 eV), with a CO stretching frequency of 2102 cm −1 (Supplementary Fig. 16a ). As reported by Tang et al. [25] , the CO adsorbed on Pt@CeDis (3) structure could react with an O atom nearby, thus creating Pt@CeO v (1) configuration. Interestingly, it was found in this study that the adsorbed CO could pull the Pt atom from the Pt–O 4 planar configuration in Pt@CeO v (1) to form CO–Pt–O 3 (Supplementary Fig. 16b , E B = −1.33 eV). The reconstruction of Pt@CeDis (3) under CO adsorption condition was demonstrated in Supplementary Fig. 17 . Moreover, the adsorption of CO on Pt@Ce2O v (1) was found rather weak ( E B = −0.07 eV). Therefore, Pt@CeDis (3) and Pt@CeO v (1) were the most possible Pt 1 /CeO 2 configurations within Pt/CeO 2 -800. Considering the lower formation energy of Pt@CeO v (1) as compared to that of Pt@CeDis (3) (Fig. 5b ), Pt@CeO v (1) should be the dominant configuration within Pt/CeO 2 -800. The formation of Pt@CeO v (1) configuration within Pt/CeO 2 -800 was also well supported by the UV–Vis spectra that Pt/CeO 2 -800 possessed higher surface structural disorder (Fig. 2c ). Based on the in situ DRIFTS results of CO adsorption showing that the CO stretching frequency on Pt/CeO 2 -550 was higher than that on Pt/CeO 2 -800, it can be concluded that Pt@CeEdge-O was the dominant configuration within Pt/CeO 2 -550, on which the adsorbed CO showed a higher stretching frequency (2047 cm −1 ) than CO-Pt@CeO v (1) within Pt/CeO 2 -800 (2022 cm −1 ). Moreover, the calculated E B of CO-Pt@CeO v (1) (−1.33 eV) was higher than that of CO-Pt@CeEdge-2O (−0.36 eV), which was well supported by the CO-TPD results showing that the CO adsorption on Pt/CeO 2 -800 catalyst was indeed stronger than that on Pt/CeO 2 -550 catalyst (Supplementary Fig. 18 ). The Bader charge analysis was conducted on Pt@CeEdge-O and Pt@CeO v (1) configurations to further evaluate the electronic structure of Pt 1 sites. As shown in Supplementary Fig. 19 , the Pt atom in Pt@CeEdge-O representing Pt/CeO 2 -550 catalyst showed a more positive Bader charge (+1.55) than that in Pt@CeO v (1) (+0.75) representing Pt/CeO 2 -800 catalyst, which could be resulted from the higher CN Pt– O of Pt atom in Pt@CeEdge-O. Such results were in consistence with XPS and XANES analysis suggesting that the Pt single atoms in Pt/CeO 2 -550 catalyst were in higher valence state than those in Pt/CeO 2 -800 catalyst. CO oxidation mechanism on Pt/CeO 2 -550 and Pt/CeO 2 -800 To understand the rationale for different CO oxidation activity on Pt/CeO 2 -550 and Pt/CeO 2 -800, the CO oxidation mechanisms on Pt@CeEdge-O and Pt@CeO v (1) were studied by DFT calculations. As shown in Fig. 6a , on Pt@CeEdge-O (the dominant configuration of Pt/CeO 2 -550), CO first picked up the O atom on top of Pt (A1) to form CO 2 that was physisorbed on the surface (A2), with a reaction energy of −3.79 eV. The CO 2 was found to desorb from the surface with a desorption energy of 0.29 eV to form Pt@CeEdge-2O configuration (A3), followed by the adsorption of O 2 on Pt atom with an adsorption energy of −0.43 eV (A4). Another CO was found to co-adsorb with O 2 on Pt atom (adsorption energy = −0.16 eV) to form A5 configuration. After a transition state of TS-A1 with an activation barrier of 0.45 eV, configuration A5 could transform into A6 (reaction energy = −0.59 eV), during which CO could pick up an O atom from the adsorbed O 2 to form CO 2 . The CO 2 subsequently desorbed from the surface with a desorption energy of −1.82 eV, resulting in the original Pt@CeEdge-O structure. Fig. 6: CO oxidation mechanisms on different Pt 1 /CeO 2 catalysts. Proposed mechanisms of CO oxidation on a Pt@CeEdge-O (representing Pt/CeO 2 -550 catalyst) and b Pt@CeO v (1) (representing Pt/CeO 2 -800 catalyst). “TS” indicates transition states. Potential energies were calculated with respect to CO and O 2 in gas phase. Full size image As shown in Fig. 6b , on Pt@CeO v (1) , CO was found to adsorb on Ce atom with an oxygen vacancy (B1) to form configuration B2, with an adsorption energy of −0.45 eV. The adsorbed CO could react with Pt to pull it up forming a CO–Pt–O 3 coordination (B3). This process was exothermic with a reaction energy of −0.81 eV and but not spontaneous with an activation barrier of 0.88 eV (TS-B1). Then, O 2 could adsorb on a Ce atom nearby (B4) with an adsorption energy of −0.50 eV. The adsorbed CO could react with a lattice O to form CO 2 (B5), with a reaction energy of −1.62 eV and an activation barrier of 1.26 eV (TS-B2). After the desorption of CO 2 (desorption energy = 0.12 eV), configuration B6 with two oxygen vacancies and adsorbed O 2 molecule was formed. O 2 could dissociate to fill these two oxygen vacancies (B7) after overcoming an activation barrier of 1.10 eV (TS-B3). Another CO could react with one of the dissociated O atoms to form a physiosorbed CO 2 molecule (B8). This step was highly exothermic with a reaction energy of −4.12 eV and the CO 2 could then desorb with a desorption energy of 0.46 eV to form original Pt@CeO v (1) structure (B1). Comparing the above two proposed mechanisms for CO oxidation, it can be concluded that the oxidation of CO required three steps with sizable activation barrier on Pt@CeO v (1) (the dominant structure on Pt/CeO 2 -800), while only one with a relatively lower barrier on Pt@CeEdge-O (the dominant structure on Pt/CeO 2 -550), well explaining why Pt/CeO 2 -800 showed markedly lower CO oxidation activity than Pt/CeO 2 -550. The results of dynamic oxygen storage capacity (OSC) test further confirmed that O 2 could be better activated and consumed by CO on Pt/CeO 2 -550 than on Pt/CeO 2 -800 (Supplementary Fig. 20 ), well supporting the DFT calculation results that the CO oxidation and O 2 dissociation (A5 → TS-A1 → A6) on Pt/CeO 2 -550 only needed to overcome much lower activation barrier comparing to those on Pt/CeO 2 -800 (B4 → TS-B2 → B5 and B6 → TS-B3 → B7). The lower apparent activation energy ( E a ) for CO oxidation on Pt/CeO 2 -550 (43 kJ∙mol −1 ) than that on Pt/CeO 2 -800 (52 kJ∙mol −1 ) (Supplementary Fig. 21 ) should also be resulted from the more efficient activation of reactants. The stability of Pt/CeO 2 -550 and Pt/CeO 2 -800 under reaction conditions was evaluated in a two-round CO oxidation activity test and through comparison to Pt cluster and nanoparticle catalysts on CeO 2 . Almost no change in CO oxidation activity was observed on both Pt/CeO 2 -550 and Pt/CeO 2 -800 during the two rounds of tests up to 500 °C (both with constantly lower activity than Pt cluster and nanoparticle catalysts) (Supplementary Fig. 22 ), suggesting the high stability of Pt 1 catalysts under CO oxidation atmosphere in this study. Considering the inevitable presence of water vapor in vehicle exhaust, the CO oxidation on both catalysts was also performed under wet condition. As shown in Supplementary Fig. 23 , Pt/CeO 2 -550 still exhibited much higher CO oxidation activity than Pt/CeO 2 -800 under wet condition. NH 3 oxidation behavior on Pt/CeO 2 -550 and Pt/CeO 2 -800 As discussed above, through simply controlling the calcination temperatures, Pt single atoms with different coordination environments were successfully constructed on CeO 2 . It has been demonstrated that Pt single atoms with a CN Pt– O of ca . 5 on Pt/CeO 2 -550 could better catalyze CO oxidation than those on Pt/CeO 2 -800 with a CN Pt– O of ca . 4. To further evaluate the catalytic performance of Pt/CeO 2 -550 and Pt/CeO 2 -800 in other oxidation reactions, NH 3 oxidation, a relatively less studied but important catalytic oxidation reaction in emission control field [53] , [54] , was selected as a probe reaction. As shown in Fig. 7 , contrary to the trend observed in CO oxidation reaction, surprisingly, Pt/CeO 2 -800 exhibited much superior NH 3 oxidation performance than Pt/CeO 2 -550. The NH 3 oxidation reaction on Pt/CeO 2 -800 even showed slightly higher N 2 selectivity than that on Pt/CeO 2 -550 especially at 350 °C (Supplementary Fig. 24 ), and such discrepancy was mainly due to the reduced formation of non-selective oxidation products including N 2 O, NO, NO 2 at high temperatures on Pt/CeO 2 -800 (Supplementary Fig. 25 ). The NH 3 oxidation activity on CeO 2 , Pt/CeO 2 -550 and Pt/CeO 2 -800 was also tested in the presence of H 2 O. After adding 5% H 2 O to the feed gas, Pt/CeO 2 -800 still exhibited better NH 3 oxidation activity than Pt/CeO 2 -550 (Supplementary Fig. 26 ). Fig. 7: NH 3 oxidation activity. NH 3 oxidation performance on Pt/CeO 2 -550 and Pt/CeO 2 -800 catalysts as well as CeO 2 support (Reaction condition: [NH 3 ] = 500 ppm, [O 2 ] = 5%, balanced with Ar, WHSV = 200,000 mL∙g cat −1 ∙h −1 ). Full size image To reveal the intrinsic reasons for the higher NH 3 oxidation activity on Pt/CeO 2 -800, NH 3 -TPD was first conducted to investigate the NH 3 adsorption capacity on pure CeO 2 support and Pt/CeO 2 catalysts (Fig. 8a ). Three NH 3 -desorption peaks at ca . 130, 170 and 220 °C were observed on Pt/CeO 2 -550 (denoted as peaks α, β, and γ) similar to those observed on CeO 2 support, which could be assigned to the desorption of NH 3 species adsorbed on CeO 2 sites and Pt sites with weak (α and β) or strong (γ) adsorption strength [55] . Interestingly, the peak γ on Pt/CeO 2 -550 showed a much higher relative intensity than that on CeO 2 support, indicating that the interaction between Pt single atoms and CeO 2 support could generate extra sites for stronger NH 3 adsorption. More importantly, on Pt/CeO 2 -800, a new intensive NH 3 -desorption peak (δ) was clearly observed, which could be attributed to NH 3 species more strongly bound to Pt single atoms or Ce atoms adjacent to Pt atoms on Pt/CeO 2 -800 with another unique coordination environment (i.e., Pt atoms substituting Ce sites at CeO 2 (110) terrace). Due to the limited NH 3 conversion below 150 °C on Pt/CeO 2 -550 and Pt/CeO 2 -800, the NH 3 oxidation activity on both catalysts should be mainly related to the NH 3 species strongly adsorbed on Pt sites (peaks γ and δ). 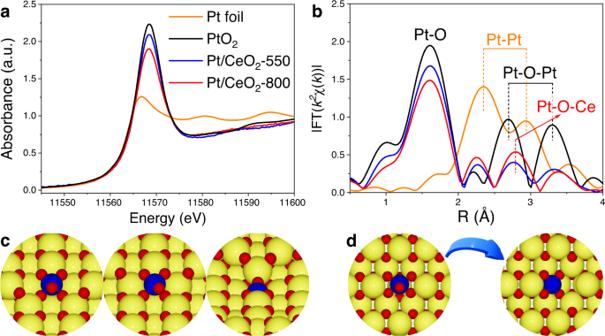Fig. 4: Coordination environment of Pt single atoms determined by XAS analysis. aNormalized XANES andbEXAFS magnitude of the Fourier transformedk2-weighted χ(k) data for Pt/CeO2-550 (blue) and Pt/CeO2-800 (red) at the Pt-L3edge. Pt foil (orange) and PtO2(black) references were used for XANES linear combination fitting and EXAFS comparison.cThree possible geometries of Pt single atoms at the edge or step sites on CeO2(110) within Pt/CeO2-550.dThe reconstruction of Pt single atoms on CeO2(110) terrace from six-coordination sites to square-planar like coordination sites within Pt/CeO2-800. As listed in Supplementary Table 4 , from the deconvolution results of NH 3 -TPD profiles, a much higher ratio of NH 3 species more strongly adsorbed on Pt sites was observed on Pt/CeO 2 -800. Given the near zero order of NH 3 in NH 3 oxidation reaction (Supplementary Fig. 27 ), the adsorption capacity of NH 3 at the investigated temperature regime would strongly determine the NH 3 oxidation activity on Pt/CeO 2 -550 and Pt/CeO 2 -800 catalysts. More strongly adsorbed NH 3 species on Pt/CeO 2 -800 catalyst could be one of the main reasons for its much higher catalytic performance in NH 3 oxidation reaction. Fig. 8: NH 3 adsorption properties of Pt 1 /CeO 2 catalysts. a NH 3 -TPD profiles on CeO 2 , Pt/CeO 2 -550, and Pt/CeO 2 -800; b in situ DRIFTS of NH 3 adsorption at 100 °C; in situ DRIFTS of NH 3 adsorption and desorption on c Pt/CeO 2 -550 and d Pt/CeO 2 -800. Full size image To further investigate the surface acidity of Pt/CeO 2 -550 and Pt/CeO 2 -800, in situ DRIFTS of NH 3 adsorption at 100 °C was conducted (Fig. 8b ). The bands at 1113, 1132, 3283 and 3364 cm −1 could be assigned to NH 3 adsorbed on Lewis acid sites. The bands at 1420 and 1680 cm −1 could be attributed to NH 4 + bound to Brønsted acid sites [55] , [56] . The other bands at 1023, 1285, 1397, 1509, 1576, and 1591 cm −1 could be assigned to nitrate species generated by the oxidation of adsorbed NH 3 [57] , [58] . Considering the same initial CeO 2 support and Pt loading of Pt/CeO 2 -550 and Pt/CeO 2 -800 catalysts, the more intensive bands of nitrates on Pt/CeO 2 -800 suggested that the adsorbed NH 3 on this catalyst could be better activated and oxidized mainly due to its unique local surface microstructure. In situ DRIFTS of NH 3 adsorption–desorption was also conducted to further evaluate the strength of surface acid sites on Pt/CeO 2 -550 and Pt/CeO 2 -800 (Fig. 8c, d ). It was clearly demonstrated that the NH 3 bands located at 1113–1132 cm −1 on Pt/CeO 2 -800 were much more intensive than those on Pt/CeO 2 -550 and also showed much higher stability in Ar flow during the temperature elevation. The formation of Pt 1 sites with different configurations on Pt/CeO 2 -550 and Pt/CeO 2 -800 should account for the distinct strength of NH 3 adsorption on these two catalysts. Based on DFT calculations, higher adsorption energy of NH 3 on Pt@CeO v (1) ( E B = −1.10 eV) was observed than on Pt@CeEdge-O ( E B = −0.73 eV) (Supplementary Fig. 28 ), further confirming this viewpoint. Besides, it was found that NH 3 could be preferentially adsorbed on Ce atoms adjacent to Pt atoms on both structures rather than on Pt single atoms directly. To evaluate the reactivity of adsorbed NH 3 on Pt/CeO 2 -550 and Pt/CeO 2 -800 catalysts, in situ DRIFTS of O 2 reacting with pre-adsorbed NH 3 at 175 °C was performed (Supplementary Fig. 29 ). As expected, more NH 3 adsorbed on Lewis acid sites (1067, 1105 and 1132 cm −1 ) were observed on Pt/CeO 2 -800 than on Pt/CeO 2 -550 at 175 °C. With the introduction of O 2 , the NH 3 species adsorbed on Brønsted acid sites (1424/1435 and 1650 cm −1 ) showed almost no reactivity. In contrast, the NH 3 species coordinated to Lewis acid sites could effectively react with O 2 , and such NH 3 species on Pt/CeO 2 -800 catalyst were consumed much faster than those on Pt/CeO 2 -550 (Supplementary Fig. 30 ). To better reveal the intrinsic reason for the higher NH 3 oxidation activity on Pt/CeO 2 -800, DFT calculations for mechanism study were also performed. It is worth noting that the overall stoichiometric reaction of NH 3 oxidation is 
    4NH_3+3O_2→ 2N_2+6H_2O
 (1) involving a number of steps, full consideration of which is beyond the scope of this work. Instead, we have resorted to consideration of the initial reaction 
    2NH_3+O_2→N_2+2H_2O+2H^∗
 (2) to provide some insights into the NH 3 oxidation process. In the above reaction, there are two H atoms (H*) remaining adsorbed on the catalyst surface after N 2 desorption. H 2 O molecules formed from the –OH groups can subsequently desorb and a surface oxygen vacancy will be created, which can be healed by the adsorption and dissociation of O 2 . More details of mechanisms and their energetics can be found in Supplementary Figs. 31 and 32 , and the simplified pictures presented in Fig. 9 capture the gist of our argument. Fig. 9: NH 3 oxidation mechanisms on different Pt 1 /CeO 2 catalysts. Proposed mechanisms of NH 3 oxidation on a Pt@CeEdge-O (representing Pt/CeO 2 -550 catalyst) and b Pt@CeO v (1) (representing Pt/CeO 2 -800 catalyst). Potential energies were calculated with respect to NH 3 and O 2 in gas phase. Full size image On Pt@CeEdge-O (Fig. 9a ), the NH 3 oxidation started with the adsorption of NH 3 on the Ce atom adjacent to Pt atom, on the upper terrace (C2). After dissociation of two N–H bonds, the resulting H atoms combined with O atom on top of Pt to form H 2 O (C3), which then desorbed from the surface leaving –NHO group behind (C4). Afterwards, the adsorption of the second NH 3 molecule on the same Ce atom could occur (C5). After the dissociation of two N–H bonds of the second NH 3 molecule and the diffusion of resulting H atoms, two –NHO groups were formed (C6), which could then react with each other to form N 2 H 2 adsorbed on the surface (C7). Subsequently, N 2 could be formed after the dissociation of the two N–H bonds (C8) and then desorbed from the surface leaving four H atoms on the catalyst (C9). The followed step was the formation and desorption of second H 2 O molecule, thus creating an oxygen vacancy (C10). The vacancy could be filled by the adsorption of O 2 (C11). After reconstruction, the original structure with the addition of two H atoms on the upper terrace was achieved (C12). A similar process was observed on Pt@CeO v (1) as well (Fig. 9b ). The oxidation of NH 3 on Pt@CeO v (1) started with the adsorption of NH 3 on the Ce atom adjacent to Pt atom with an oxygen vacancy (D2), followed by the co-adsorption of O 2 to form D3 configuration. After the dissociation of two N–H bonds and O 2 molecule, a H 2 O molecule was formed (D4), which could desorb from surface leaving –NHO group behind (D5). Then, the second NH 3 molecule could adsorb on another Ce atom nearby the Pt atom (D6). After the dissociation of two N–H bonds of the second NH 3 molecule, two –NHO groups were formed on Pt@CeO v (1) (D7). The two H atoms from these two –NHO groups could recombine with surface O atom to form second H 2 O (D8), which could desorb from surface leaving two –NO groups and an oxygen vacancy (D9). The formed N 2 from these two –NO groups could then desorb from surface (D10). After a surface structural reconstruction, the catalyst could return to its starting configuration with two additional H atoms on the terrace of the CeO 2 (110) surface (D11). When comparing the two reaction mechanisms mentioned-above, it can be observed that the N atoms in –NHO or –NO groups on Pt@CeO v (1) (representing Pt/CeO 2 -800 catalyst) were coordinated to Pt atom, which could weaken the strength of Pt–O bond and accordingly facilitate the formation (D7 → D8) and desorption (D8 → D9) of the second H 2 O molecule. The desorption energy of the second H 2 O formed on Pt@CeO v (1) was determined as 1.19 eV, much lower than that on Pt@CeEdge-O representing Pt/CeO 2 -550 catalyst (2.31 eV) on which the N atoms in –NHO or –NO groups were coordinated to Ce atoms. For the NH 3 oxidation on both Pt@CeEdge-O and Pt@CeO v (1) , the desorption of the second H 2 O molecule (C9 → C10 and D8 → D9, respectively) was the rate limiting step. Therefore, the lower desorption energy of the second H 2 O molecule on Pt@CeO v (1) was one of the main reasons for the much higher NH 3 oxidation activity obtained on Pt/CeO 2 -800. Pt single atom catalysts with different local coordination environments on CeO 2 support were finely fabricated by a simple calcination temperature control strategy. With the calcination temperature increased from 350 to 800 °C, the Pt clusters could first disperse into Pt single atoms, and then the Pt single atoms with much stronger interaction with CeO 2 through Pt–O–Ce linkages were created. 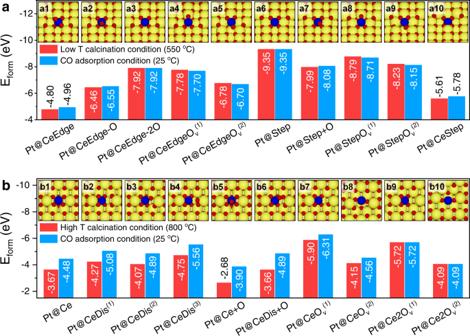Fig. 5: Determination of Pt1configurations on CeO2through DFT calculations. The formation energy (Eform) of the considered Pt1configurations on CeO2(110) under different conditions, i.e., low-temperature (Low T) calcination condition (550 °C, 0.21 atm O2pressure), high-temperature (High T) calcination condition (800 °C, 0.21 atm O2pressure), and CO adsorption condition (25 °C, 10−20atm O2pressure) withinaPt/CeO2-550 andbPt/CeO2-800. The insert figures are the top view of considered configurations of isolated Pt atoms at or near the edge/step sites on CeO2(110) surface within Pt/CeO2-550 (a1−10), and at the Ce substitution sites of CeO2(110) surface within Pt/CeO2-800 (b1−10). Large yellow, medium blue, and small red balls represented Ce, Pt, and O atoms. Different from Pt/CeO 2 -550 catalyst in which the Pt single atoms were mainly located at the edge sites of CeO 2 support, for Pt/CeO 2 -800 catalyst, the Pt single atoms were mainly incorporated into the surface lattice of CeO 2 with further structural reconstruction to form a square-planar like coordination environment on CeO 2 terrace. Although the Pt single atoms on Pt/CeO 2 -800 catalyst showed rather limited catalytic activity in CO oxidation reaction due to its inferior ability to activate O 2 , the enhanced surface acidity for NH 3 adsorption/activation and the easier desorption of H 2 O produced during the reaction enabled Pt/CeO 2 -800 to exhibit much higher NH 3 oxidation activity than that on Pt/CeO 2 -550. It is suggested that the precise control of the coordination environments of Pt single atoms is beneficial for maximizing their catalytic performance in different oxidation reactions. This work can provide instructive insights into the flexible tuning of local coordination environments of single atom catalysts for more efficient application in different target reactions. Catalyst preparation Before being used as a support, commercial CeO 2 (high surface area ceria with the BET surface area as ca . 120 m 2 /g) was pre-calcined in air at 800 °C for 12 h to minimize its potential structural changes in the subsequent catalyst preparation process. To prepare CeO 2 supported Pt catalysts, 1.00 wt.% Pt using Pt(NO 3 ) 2 as precursor was loaded onto the pretreated CeO 2 support by incipient wetness impregnation (IWI) method. After impregnation of Pt(NO 3 ) 2 onto CeO 2 , the wet powder was dried in air at 120 °C for 1 h. Afterwards, the obtained powder was calcined in air at 350, 550, 700, or 800 °C for 2 h. The obtained catalysts were denoted as Pt/CeO 2 -X, with X °C as calcination temperature. The practical mass loadings of Pt in the selected catalysts were determined by inductively coupled plasma-optical emission spectrometry (ICP-OES). As expected, Pt/CeO 2 -550 (0.92 wt.%) and Pt/CeO 2 -800 (0.90 wt.%) showed almost the same Pt loadings, which were very close to the nominal Pt loading (1.00 wt.%). Characterizations The specific surface area and pore volume were measured by N 2 physisorption at −196 °C using a Micromeritics ASAP-2020 analyzer. Before each test, the samples were degassed at 300 °C for 4 h. The specific surface area was calculated using Brunauer-Emmett-Teller method, and the pore volume and pore size distribution were determined by BJH method using the desorption isotherms. In situ diffuse reflectance infrared Fourier transform spectroscopy (in situ DRIFTS) study was carried out on a Thermo Nicolet iS50 FTIR spectrometer equipped with a liquid nitrogen-cooled mercury–cadmium–telluride (MCT) detector. In each test, 50 mg of catalyst powder was placed in the DRIFTS cell (PIKE Technologies DiffusIR), pressed, and mounted. The catalysts were first pretreated in air at 300 °C for 1 h. Afterwards, the catalysts were cooled down step-wise to room temperature. During this process, the background spectra were collected at target temperatures for different experiments (e.g., 25 °C for CO adsorption, 25 °C for methanol adsorption, 100/125/150/175/200/225/250 °C for NH 3 adsorption/desorption, and 175 °C for NH 3 oxidation). For CO adsorption, methanol adsorption, or NH 3 adsorption/desorption/oxidation experiments, the feed gas consisted of 1% CO, 15% methanol, or 500 ppm NH 3 and/or 5 vol% O 2 (when used), respectively, using Ar as balance. The total flow rate was controlled at 83.33 mL∙min −1 . All the spectra were collected from 400 to 4000 cm −1 at a resolution of 4 cm −1 for 100 scans. H 2 -temperature-programmed reduction (H 2 -TPR) was conducted on a Quantachrome Autosorb-iQ instrument. Typically, 30 mg of sample was loaded in a U-type quartz tube reactor and pretreated with air at 400 °C for 1 h. When the sample was cooled down to room temperature in air, the feeding gas was switched to 10 vol% H 2 balanced with Ar (30 mL∙min −1 ). Then, the reactor was heated linearly to 900 °C with a ramping rate of 10 °C∙min −1 . The signal of H 2 consumption was monitored by a thermal conductivity detector (TCD). H 2 O moisture in the gas mixture was removed by a cold trap filled with liquid N 2 before passing into the TCD. Ultraviolet-visible (UV–Vis) spectra were collected on a Shimadzu UV-2401 PC instrument in diffuse mode. BaSO 4 was used as a reference and the spectra collection range was 200−800 nm. Samples were exposed to air at room temperature throughout the experiments. Atomic-resolution aberration-corrected high angle annular dark field scanning transmission electron microscopic (AC-HAADF-STEM) images were collected on a FEI Titan Cubed G2 60-300 aberration-corrected S/TEM instrument at 300 kV accelerating voltage. The observations were performed in the HAADF mode, which allowed Z-contrast imaging. The probe convergence angle on the Titan electron microscope was 22 mrad, and the angular range of the HAADF detector was from 79.5 to 200 mrad. To prepare the TEM samples, an appropriate amount of sample powder was dispersed in ethanol and then dropped on a 3 mm TEM Mo grid. The images of energy dispersive spectroscopy (EDS) elemental mapping in the STEM mode were obtained from the Titan electron microscope using SuperX system. In situ XRD experiments were conducted on a Rigaku SmartLab SE XRD instrument equipped with a high speed 1D silicon strip detector (D/teX Ultra 250, Rigaku, Japan) and an in situ cell (Reactor X, Rigaku, Japan). X-rays were generated from a Cu source, with a tube operational power of 2.2 kW (Cu Kα). Additional PXRD parameters were as follows: goniometer radius = 300 mm, incident and receiving Soller slits = 2.5 °, length limiting slit = 10 mm, with a receiving slit Ni filter mitigating the Cu Kβ signal. The temperature of the sample was controlled by IR heating of the quartz sample holder (sample indention dimensions: 13 × 20 × 0.4 mm) from below, and the gas composition in the cell was controlled by a bank of mass flow controllers (Brooks 5850e, Brooks Instrument, Hatfield, PA, USA). 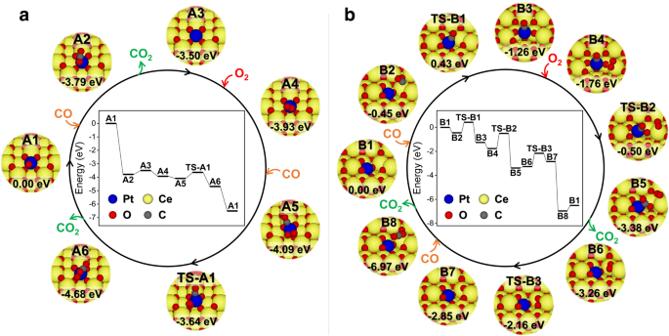Fig. 6: CO oxidation mechanisms on different Pt1/CeO2catalysts. Proposed mechanisms of CO oxidation onaPt@CeEdge-O (representing Pt/CeO2-550 catalyst) andbPt@CeOv(1)(representing Pt/CeO2-800 catalyst). “TS” indicates transition states. Potential energies were calculated with respect to CO and O2in gas phase. During the experiments, dry air flowed through the in situ cell (100 mL∙min −1 ). Samples were held on at 25 °C for 5 min, and then the XRD scans were performed continuously throughout the temperature ramping, holding and cooling steps. In more detail, the samples were heated from 25 °C to the target temperatures (550 or 800 °C) with a ramping rate of 2 °C∙min −1 , held at the target temperatures (550 or 800 °C) for 2 h, and finally cooled to 25 °C at a rate of 2 °C∙min −1 . The XRD scans were taken from 25 to 50° at a scan rate of 2 °C∙min −1 , with a step size of 0.01°. ICP-OES measurement was conducted on an Optima 8300 instrument (PerkinElmer). The incident power was set at 13,000 W and the wavelength for Pt detection was 265.945 nm. XAS for Pt L 3 -edge in fluorescence mode was measured at beamline 7-BM QAS of the National Synchrotron Light Source II (NSLS-II) at Brookhaven National Laboratory. The energy range of the X-ray provided by this beamline was 4.7–31 keV. Its monochromator is equipped with a Si(111) channel-cut crystal and runs at continuous scan mode. The duration of a typical scan was 30 s and each sample was scanned 40 times. Samples were exposed to air at room temperature throughout the experiments. The XAS data including X-ray absorption near edge structure (XANES) and extended X-ray absorption fine structure (EXAFS) were analyzed using Demeter software package. X-ray photoelectron spectroscopy (XPS) was collected on a VG CLAM 4 MCD analyzer. Before the analysis, the samples were degassed in a preparation chamber (10 −5 Torr) for 0.5 h. Then, the samples were put into the analysis chamber (3 × 10 −9 Torr) for further analysis. The binding energies (BE) were calibrated with C1s line at 284.6 eV. Raman spectra were collected on a Renishaw Laser Raman spectrometer (Renishanplc) with an Ar + laser beam. The emission line was 532 nm and the output power was 10 mW. Samples were exposed to air at room temperature throughout the experiments. CO-temperature programmed desorption (CO-TPD) was conducted in a fixed-bed quartz tube flow reactor with an online mass spectrometer (Hiden Analytical, HPR20 R&D). The mass-to-charge ratio ( m / z ) of 28 was used to monitor CO. In each test, 100 mg sample was pretreated by air at 300 °C for 1 h and then saturated with CO at 30 °C. Then, Ar was introduced into the quartz tube reactor to remove the weakly adsorbed CO. Finally, the sample was heated linearly to 300 °C at a rate of 10 °C∙min −1 in flowing Ar. The dynamic oxygen storage capacity (OSC) was measured by a multi-pulse experiment under alternating pulses of 2% CO/4% O 2 with a total flow rate of 100 mL∙min −1 . Before testing, all samples were pretreated in air at 300 °C for 1 h. A single cycle lasted 1 min, with 30 s CO/30 s O 2 cycling switch controlled by automatic mass flow controller (MFC) systems. The OSC values were calculated from the averaged CO 2 formation in a cycle (30 s + 30 s) detected by an online mass spectrometer (Hiden Analytical, HPR20 R&D). NH 3 -temperature-programmed desorption (NH 3 -TPD) was carried out in a fixed-bed quartz flow reactor connected with an online Thermo Nicolet iS10 FTIR spectrometer equipped with a 2 m path-length gas cell (200 mL volume). In each test, 100 mg sample was pretreated by pure Ar at 200 °C for 1 h and then saturated with NH 3 at 100 °C. Then, Ar was introduced into the quartz tube reactor again to remove the weakly adsorbed NH 3 . Finally, the sample was heated linearly to 500 °C at a rate of 10 °C∙min −1 in the flowing Ar (100 mL∙min −1 ). Details of density functional theory (DFT) based calculations DFT calculations were performed using the Vienna ab initio Simulation Package (VASP) [59] , employing the projector-augmented wave (PAW) [60] , [61] and plane-wave basis set. The generalized-gradient approximation (GGA) was used in the form of the Perdew-Burke-Ernzerhof (PBE) [62] functional together with the DFT-D3 correction [63] to describe electronic exchange-correlation. The DFT + U method with U = 5 eV for Ce 5f orbitals [64] was used to properly describe the electronic structure of CeO 2 . The electron kinetic energy cut-off for plane-wave expansion was set to 500 eV. For modeling the CeO 2 (110) surface, a 5 layer 4 × 3 CeO 2 (110) slab was constructed, i.e., 12 Ce and 24 O atoms per layer, using the optimized lattice constant of 5.479 Å. For modeling the stepped CeO 2 (110) surface, a twice-large slab was removed with half of the top CeO 2 layer to create the step. 15 Å vacuum added along the surface normal direction was used to decouple periodical images along the surface normal direction. Given the large size of the supercell, the Brillouin zone was sampled with one point at the zone center, using a Gaussian smearing with σ = 0.1 eV for structural relaxation. All electronic cycles converged to 10 −5 eV. All structures were relaxed to minimize the stress until all components of forces acting on each atom were less than 10 −2 eV/Å. To search the preferable location of Pt atom on surface, various surface Ce atoms were replaced with Pt atoms. To mimic the cases that Pt atom was next to O-vacancies, one or two O atoms nearby Pt were removed to create a scenario. To mimic the cases that Pt atom was coordinated with 5 or 6 O atoms, one O atom was added on top of Pt. For step surface, Pt atoms adsorbed at the step sites were also considered. To evaluate the relative formation energy of Pt 1 configurations, the formation energy of Pt 1 /CeO 2 was defined as 
    E_form=F_Pt_1/CeO_2-F_CeO_2,
 (3) where \({F}_{{{{{{{\rm{Pt}}}}}}}_{1}/{{{{{\rm{CeO}}}}}}_{2}}\) and \({F}_{{{{{{\rm{CeO}}}}}}_{2}}\) were the free energy of Pt 1 /CeO 2 system and CeO 2 surface. The free energy of a system was defined as 
    F=E+F_Vib+PV-N_Ceμ_Ce^o-N_Oμ_O-N_Ptμ_Pt,
 (4) where \(E\) , \({F}_{{{{{{\rm{Vib}}}}}}}\) , and \({PV}\) were the total energy (calculated from DFT), the vibrational contribution to free energy, and the contribution to free energy of the change of pressure and volume, respectively. The difference between \({PV}\) term of Pt 1 /CeO 2 and clean CeO 2 surface was small and could be ignored. In this work, the difference in \({F}_{{{{{{\rm{Vib}}}}}}}\) between Pt 1 /CeO 2 and clean CeO 2 surface was not included for computational feasibility, as 20 Pt 1 /CeO 2 configurations with large simulation supercell were considered. Nevertheless, such contribution was expected to play a minor role because of the large difference between the formation energy of considered Pt 1 /CeO 2 configurations, as shall be seen. \({N}_{X}\) and \({\mu }_{X}\) were the number of X atoms in the considered system and chemical potential of X atom ( X = Ce, O, or Pt), respectively. As Ce was in equilibrium with Ce atoms in bulk CeO 2 (i.e., if Ce atoms moved away from the surface, they would go to bulk CeO 2 ), \({\mu }_{{{{{{\rm{Ce}}}}}}}\) and \({\mu }_{{{{{\rm{O}}}}}}\) were not independent and 
    μ_Ce+2μ_O=E_CeO_2,
 (5) where \({E}_{{{{{{{\rm{CeO}}}}}}}_{2}}\) was the total energy per bulk CeO 2 unit. As oxygen was in equilibrium with the O 2 reservoir surrounding the surface, the chemical potential of oxygen at temperature \(\it {{{{T}}}}\) and partial pressure \({p}_{{{{{{\rm{O}}}}}}_{2}}\) was calculated as 
    μ_O(T,p)=1/2(E_Tot^O_2+E_ZPE^O_2)+μ̃_O(T,p^o)+1/2k_BT ln(p_O_2/p^o),
 (6) where \({E}_{{{{{\rm{Tot}}}}}}^{{{{{{\rm{O}}}}}}_{2}}\) and \({E}_{{{{{\rm{ZPE}}}}}}^{{{{{{\rm{O}}}}}}_{2}}\) were the total energy and zero point energy of an O 2 molecule calculated with DFT, \({k}_{B}\) was Boltzmann constant, \({p}^{o}\) was a reference pressure, and \({\tilde{\mu }}_{O}(T,{p}^{o})\) was the temperature dependent part that could be calculated from experimental data [65] , [66] . As Pt was often deposited on the surface at the beginning of the calcination process, there was no reservoir for Pt during or after calcination, thus the chemical potential of Pt was approximated as the total energy of the isolated Pt atom. The adsorption energy of CO on Pt 1 /CeO 2 was calculated as 
    E_Ads=E_CO-Pt_1/CeO_2 - E_Pt_1/CeO_2 - E_CO,
 (7) where \({E}_{{{{{{\rm{CO}}}}}}-{{{{{{\rm{Pt}}}}}}}_{1}/{{{{{\rm{Ce}}}}}}{{{{{\rm{O}}}}}}_{2}}\) , \({E}_{{{{{{{\rm{Pt}}}}}}}_{1}/{{{{{\rm{Ce}}}}}}{{{{{\rm{O}}}}}}_{2}}\) and \({E}_{{{{{{\rm{CO}}}}}}}\) were the total energy of CO adsorption configuration, Pt 1 /CeO 2 system, and an isolated CO molecule which was evaluated inside a cubic 15 × 15 × 15 Å 3 box, respectively. CO stretching frequencies were calculated using the finite-difference method as implemented in the Phonopy code (a 0.01 Å displacement was used, and electronic cycles were converged to 10 −6 eV) [67] . 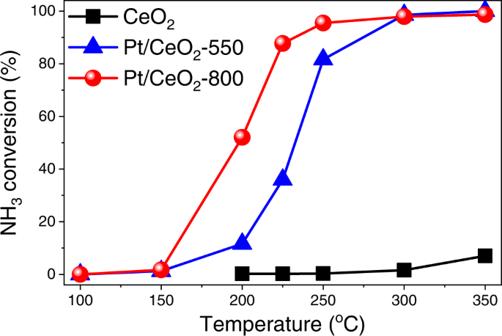Fig. 7: NH3oxidation activity. NH3oxidation performance on Pt/CeO2-550 and Pt/CeO2-800 catalysts as well as CeO2support (Reaction condition: [NH3] = 500 ppm, [O2] = 5%, balanced with Ar, WHSV = 200,000 mL∙gcat−1∙h−1). It was found that displacements applied to about 30 atoms around the adsorbed CO molecule were sufficient to obtain converged CO stretching frequencies. Since the study here involved considerations of a large number of configurations of adsorbed reactants and their intermediates as appropriate for CO oxidation and NH 3 oxidation on Pt@CeO v (1) and Pt@CeEdge-O, for computational feasibility, a CeO 2 (110) slab with 4 layers of 4 × 3 CeO 2 (110), i.e., 12 Ce and 24 O atoms per layer, was used for the investigations on Pt@CeO v (1) . A CeO 2 (110) slab with 5 layers of 1 × 3 CeO 2 (230) stepped surface, i.e., 12 Ce and 24 O atoms per layer, was used for CO oxidation study on Pt@CeEdge-O. A CeO 2 (110) slab with 4 layers of 6 × 3 CeO 2 (110) with 50% of the top layer removed, creating the step in the Pt@CeEdge-O model, was used for NH 3 oxidation study. Transition state (TS) for a reaction was determined using the nudged-elastic band (NEB) and the climbing-image (CI-) NEB methods [68] , [69] . Catalytic activity test The CO oxidation and NH 3 oxidation activities of the catalysts were evaluated in a fixed-bed quartz tube reactor. 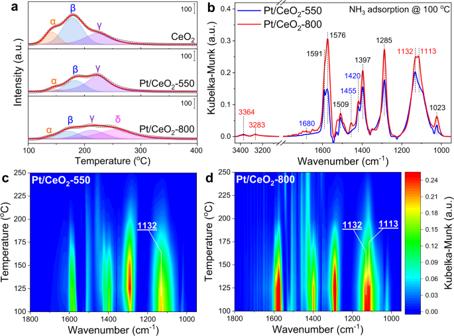Fig. 8: NH3adsorption properties of Pt1/CeO2catalysts. aNH3-TPD profiles on CeO2, Pt/CeO2-550, and Pt/CeO2-800;bin situ DRIFTS of NH3adsorption at 100 °C; in situ DRIFTS of NH3adsorption and desorption oncPt/CeO2-550 anddPt/CeO2-800. 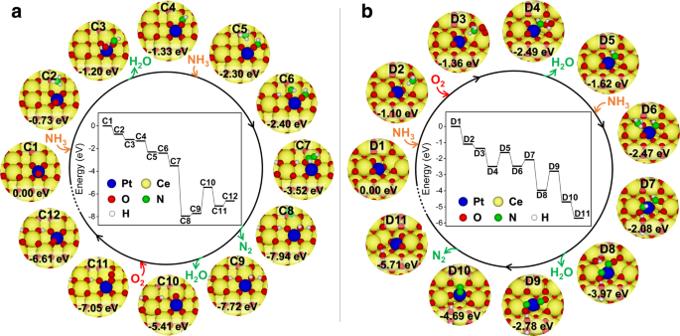Fig. 9: NH3oxidation mechanisms on different Pt1/CeO2catalysts. Proposed mechanisms of NH3oxidation onaPt@CeEdge-O (representing Pt/CeO2-550 catalyst) andbPt@CeOv(1)(representing Pt/CeO2-800 catalyst). Potential energies were calculated with respect to NH3and O2in gas phase. Samples (40–60 mesh) were mixed with SiC to minimize the heat effect (with a mass ratio of 1:10). For CO oxidation activity test, the reactants consisted of 1% CO, 1% O 2 and 5% H 2 O (if used) in Ar balance. The total flow rate was 83.33 mL∙min −1 with a weight hourly space velocity (WHSV) of 400,000 mL∙g cat −1 ·h −1 . The outlet gas was detected by an online mass spectrometer (Hiden Analytical, HPR20 R&D). The mass-to-charge ratio ( m / z ) of 28 and 44 were used to monitor CO and CO 2 , respectively. For NH 3 oxidation activity test, the reactants consisted of 500 ppm NH 3 , 5% O 2 , and 5% H 2 O (if used) in Ar balance. The WHSV was controlled at 200,000 mL∙g cat −1 ·h −1 . The concentrations of NH 3 , NO, NO 2 , and N 2 O in the outlet gas were measured by Thermo Nicolet iS10 FTIR spectrometer equipped with a 2 m path-length gas cell with 200 mL volume. All reactions were performed under steady state conditions. The CO conversion in CO oxidation reaction, and the NH 3 conversion and N 2 selectivity in NH 3 oxidation reaction were determined according to the following equations: 
    CO conversion  (%)={([CO]_in-[CO]_out)/[CO]_in}× 100%
 (8) 
    NH_3 conversion  (%)={([NH_3]_in-[NH_3]_out)/[NH_3]_in}× 100%
 (9) 
    N_2 selectivity  (%)={1-([NO]_out+[NO_2]_out+2[N_2O]_out)/([NH_3]_in-[NH_3]_out)}× 100%
 (10) In the reaction kinetics study, to avoid the heat and mass transfer effects, the reaction rates were determined with CO or NH 3 conversions below 15%, and samples (40–60 mesh) were mixed with SiC to minimize the heat effect (with a mass ratio of 1:20) before the test. For CO oxidation reaction, the feed gas consisted of 1% CO and 1% O 2 in Ar balance. The WHSV was controlled at 800,000 mL∙g cat −1 ·h −1 and 400,000 mL∙g cat −1 ·h −1 for Pt/CeO 2 −550 and Pt/CeO 2 −800, respectively. For NH 3 oxidation reaction, the feed gas consisted of 500 ppm NH 3 and 5% O 2 in Ar balance, with a WHSV of 600,000 mL∙g cat −1 ·h −1 .